Solid-source growth and atomic-scale characterization of graphene on Ag(111) Silver is a desirable platform for graphene growth because of the potential for hybrid graphene plasmonics and its emerging role as a preferred growth substrate for other two-dimensional materials, such as silicene. Here we demonstrate the direct growth of monolayer graphene on a single-crystal Ag(111) substrate. The inert nature of Ag has made it difficult to use for graphene synthesis using standard chemical vapour deposition techniques, which we have overcome by using an elemental carbon source. Atomic-scale scanning tunnelling microscopy reveals that the atomically clean graphene–silver substrate is free of organic residue and other contaminants. The dendritic graphene possesses a variety of edge terminations, many of which give rise to quantum interferences previously seen only on insulating substrates. This scattering supports spectroscopic evidence that the graphene electronic structure is minimally perturbed by the underlying silver, providing a new system in which graphene is decoupled from its growth substrate. Graphene exhibits well-known mechanical, thermal, electronic and optical properties that distinguish it from nearly all three-dimensional (3D) materials, thus motivating significant research in recent years [1] . To date, this research has primarily focused on the rich physics underlying graphene’s properties; however, current attention has shifted to interfacing graphene with alternate materials, many of which are also two-dimensional (2D), for new physics and device applications [2] , [3] , [4] . For example, hexagonal boron nitride substrates enable significant enhancements in electron mobility for graphene electronics [5] . Alternatively, integrated graphene plasmonics based on graphene interfaces with noble metals have realized architectures capable of extreme light concentration and manipulation, highly efficient photoconversion and single-molecule detection [6] , [7] . However, these interfaces are often prepared with and studied after significant material processing that contaminates the interface with a wide range of organic/inorganic species, thus compromising graphene’s intrinsic characteristics [8] , [9] . The direct growth of graphene at the desired interface provides a means to circumvent these issues and enables the fabrication of clean, well-defined interfaces. Furthermore, experiments conducted under ultra-high vacuum (UHV) permit the pristine and atomic-scale characterization of these systems, which enables elucidation of their intrinsic properties [10] . Graphene on Ag is an attractive system for these studies because of its excellent plasmonic characteristics and common use in printed electronics [11] , [12] . Even more compelling is the fact that Ag substrates have become a critical platform for novel 2D materials such as silicene, the silicon-based analogue to graphene, which has been prepared in UHV almost exclusively on Ag(111) [13] , [14] . Here we report the growth of monolayer graphene on atomically pristine single-crystal Ag(111). Growth is accomplished by evaporating atomic carbon onto a Ag(111) surface at elevated temperatures under UHV conditions. The resulting graphene is examined at the atomic scale in situ via scanning tunnelling microscopy (STM) and scanning tunnelling spectroscopy (STS), and then further characterized via ex-situ Raman spectroscopy, scanning electron microscopy and X-ray photoelectron spectroscopy (XPS). Growth occurs at relatively low temperature compared with conventional chemical vapour deposition (CVD) techniques [15] , [16] , [17] , which suggests opportunities for integrating graphene with other low-melting-point substrates. The resulting graphene demonstrates electronic independence from the Ag substrate, as seen in STS. Furthermore, the mixed graphene edges give rise to quantum interferences, which are confined to the C–C bonds, further corroborating the minimal effect of the Ag substrate on the electronic structure of the graphene [18] , [19] . 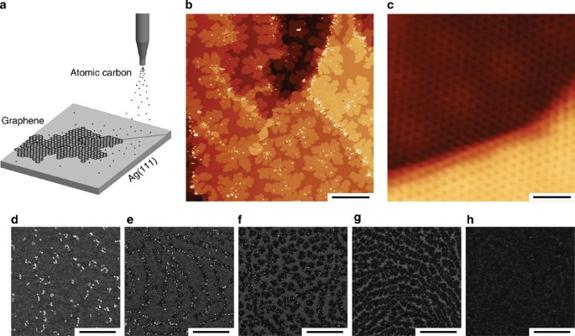Figure 1: Graphene on Ag(111). (a) Schematic of the growth process. (b) STM image of the resulting graphene morphology (scale bar, 100 nm,V=1 V,I=1 nA). (c) Atomic-resolution image of the graphene lattice across a Ag step (scale bar, 1 nm,V=25 mV,I=15 nA). (d) Scanning electron microscopy (SEM) images after growth taken in regions with increasing carbon concentration from (d–h) with a full monolayer shown inh(scale bar, 500 nm in all SEM images). Graphene growth morphology Figure 1a shows a schematic representation of the growth process, depicting the carbon evaporation, surface diffusion and initial graphene growth. The atomic carbon is deposited from a graphite rod in a manner similar to molecular beam epitaxy, where the deposition rates are estimated to be on the order of 0.1 ML min −1 . Figure 1b shows a 500 nm × 500 nm STM image of the Ag(111) surface after carbon deposition and graphene growth. The dendritic features emanating from the step edges and seen on the terraces are confirmed via atomic-resolution imaging ( Fig. 1c ) and STS measurements as graphene. Ex-situ scanning electron microscopy ( Fig. 1d–h ) can also be used to image the graphene coverage on the sample because of contrast arising from environmental degradation of the Ag(111) surface that reduces its electrical conductivity. Graphene (darker regions) is shown at full monolayer coverage in Fig. 1h . Figure 1: Graphene on Ag(111). ( a ) Schematic of the growth process. ( b ) STM image of the resulting graphene morphology (scale bar, 100 nm, V =1 V, I =1 nA). ( c ) Atomic-resolution image of the graphene lattice across a Ag step (scale bar, 1 nm, V =25 mV, I =15 nA). ( d ) Scanning electron microscopy (SEM) images after growth taken in regions with increasing carbon concentration from ( d – h ) with a full monolayer shown in h (scale bar, 500 nm in all SEM images). Full size image It is well known that low C solubility in Cu is an indicator of weak atomic interactions in the Cu–C system; therefore, graphene growth on Cu has been understood and modelled by the diffusion of C species on Cu surfaces [20] , [21] . The comparably low solubility of C in Ag [22] suggests that graphene growth on Ag(111) should follow a similar mechanism. The dendritic graphene growth is accompanied by small nanoparticles (<10 nm) of varying density and morphology on the Ag(111) surface as seen in Fig. 1b,d . The progression in Fig. 1d–h is obtained after growth at several points on the surface along a gradient in the carbon concentration, which resulted from the line-of-sight deposition. The graphene coverage increases with carbon concentration, as seen in Fig. 1d–h . The clusters that accompany graphene growth are difficult to characterize electronically because of their relatively high aspect ratios; however, atomically resolved images suggest that the graphene lattice extends over the top of the clusters ( Supplementary Fig. S1 ). The observed graphene lattice, in addition to the centralized location of the clusters within the graphene domains, suggests that the clusters could be the nucleation points for graphene growth. Furthermore, the observation of similar clustering on Cu(111) ( Supplementary Fig. S1e,f ) indicates that the clusters are likely to be carbon-based and the growth behaviour is characteristic of the deposition method. Graphene nucleation after coalescence of carbon clusters has been discussed for graphene growth on Ru substrates [23] and observed on Rh(111) [24] ; however, the clusters are generally much smaller than the ones observed here. Furthermore, the cluster morphology exhibits significant temperature dependence, which has been used to reduce their density via post-growth annealing ( Supplementary Fig. S2 ). Regardless of the exact nature of the nucleation, graphene growth is observed to originate both at atomic steps and on atomically flat terraces. 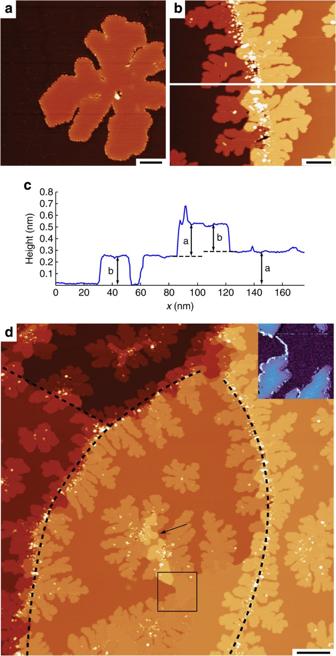Figure 2: Graphene growth morphology. (a) Growth of a graphene flake on an atomically flat terrace (scale bar, 10 nm,V=−600 mV,I=2 nA). (b) Bidirectional growth of graphene from a Ag step edge (scale bar, 15 nm,V=1 V,I=1 nA). (c) Linear topography profile along the white line inb, with the graphene–Ag step labelled b and the Ag step labelled a. (d) Characteristic STM image of the growth morphology illustrating step and terrace nucleation (scale bar, 50 nm,V=1 V,I=1 nA). Boxed region (topography) and inset (dI/dV) show a region where Ag atoms arrange at the edge of graphene growth with graphene appearing bright in the inset. The arrow indicates a region of graphene growing on a Ag island on the terrace. Figure 2a depicts the growth of graphene on an atomically flat terrace, in which graphene apparently grows outwards from a central particle(s)/nucleation point in a dendritic fashion. In general, the shape of the growth front is both temperature and carbon flux dependent, but demonstrates no repeated symmetry. In a different growth mode, graphene is observed to nucleate at the Ag step edges, shown in detail in Fig. 2b and highlighted with dashed lines in Fig. 2d . Graphene growing from the Ag step edges generally causes significant deformation of the original Ag step. Although the cause of this deformation is difficult to isolate, it is plausible that the graphene restructured the steps during growth similar to etching or restructuring of metal steps during graphene growth on Au and Rh, although this etching generally results in graphene terminating at the metal steps [25] , [26] . A linear topography profile across the graphene-covered step in Fig. 2b illustrates two major discontinuous features: a step at the interface between graphene and Ag (labelled b) and a step from one atomic terrace to another on the Ag crystal (labelled a). Although a matches well with expectations, b is somewhat smaller (~2 Å) than the expected 3.3 Å at equilibrium [27] ; however, it is difficult to draw conclusions from this fact, because this height can be affected by differences in tunnelling conductance between the two materials (seen in the STM topography data in Supplementary Fig. S3a–d ). Furthermore, graphene is also observed to grow continuously across Ag step edges ( Fig. 1c ). Figure 2: Graphene growth morphology. ( a ) Growth of a graphene flake on an atomically flat terrace (scale bar, 10 nm, V =−600 mV, I =2 nA). ( b ) Bidirectional growth of graphene from a Ag step edge (scale bar, 15 nm, V =1 V, I =1 nA). ( c ) Linear topography profile along the white line in b , with the graphene–Ag step labelled b and the Ag step labelled a. ( d ) Characteristic STM image of the growth morphology illustrating step and terrace nucleation (scale bar, 50 nm, V =1 V, I =1 nA). Boxed region (topography) and inset ( dI / dV ) show a region where Ag atoms arrange at the edge of graphene growth with graphene appearing bright in the inset. The arrow indicates a region of graphene growing on a Ag island on the terrace. Full size image All graphene presented in this work was electronically confirmed with STS as a single layer. Although raised regions of growth appear at some terrace nucleation sites (indicated in Fig. 2d ), STS data (inset Fig. 2d ) demonstrate the electrical homogeneity of the upper and lower graphene (light blue), and its stark contrast to Ag (purple). Noting that the height difference between the two graphene regions is approximately the measured height of a Ag step, it appears that the raised graphene is growing on top of a Ag island on the terrace. Similar islands were observed to border graphene edges (see Fig. 1b ) and growth on top of these islands would explain the electronic signature of monolayer graphene. The presence of monolayer graphene is also suggested by the symmetric 2D band (full width at half maximum (FWHM)=42 cm −1 ) in the Raman data [28] . As seen in other studies, the growth of graphene from atomic carbon is not self-limiting [29] , [30] , [31] , with large one-dimensional objects appearing at higher coverages ( Supplementary Fig. S4c ). Supplementary Fig. S4b illustrates that these features are the result of colliding growth fronts of graphene flakes, which grow vertically (off of the surface) after meeting. These large features are likely to account for much of the roughness and disorder often seen in atomic source growth [31] . Ex-situ spectroscopy The Raman spectrum in Fig. 3a shows the commonly observed D (~1,350 cm −1 ), G (~1,589 cm −1 ) and 2D (~2,690 cm −1 ) peaks for graphene [32] . In addition, the spectrum includes peaks at 1,625 and 2,940 cm −1 , which are attributed to the defect-related D ′ band and the D + G band, respectively [28] . The prominent D band and the appearance of the D ′ and D + G bands are generally related to point defects in the basal plane or edges of single-crystalline graphene domains [33] . We use two metrics from recent studies to suggest that the defect-related peaks observed in Fig. 3d are related to the high density of graphene boundaries in the observed growth process. First, the FWHM of the D band is ~25 cm −1 . A study on graphene nanoribbons (GNRs) has shown that the I ( D )/ I ( G ) ratio scales with the GNR width, but that the FWHM of the D band, is constant and generally <30 cm −1 if the basal plane of the GNR is unperturbed [34] . Second, the I ( D )/ I ( D ′) ratio of ~4 has been linked to a higher concentration of edge defects as opposed to vacancies or sp 3 carbon in the basal plane [35] . Noting that the laser spot size is ~2–3 μm ( Fig. 2d is 500 nm × 500 nm or approximately an order of magnitude smaller in area), it is clear that the proportion of edges is much larger than graphene grown by CVD methods on Cu [36] . Furthermore, common STM observation of standing waves at mixed/armchair edges in the dendritic graphene indicates that a large portion of the edges are capable of supporting the intervalley scattering process associated with the presence of the Raman D band [37] . The STM images also corroborate the lack of point defects on the basal plane, which are easily spotted because of their strong electronic scattering signatures [38] . 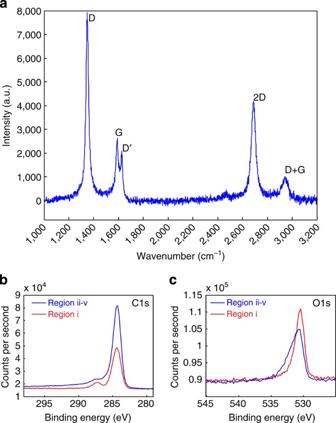Figure 3: Large-scaleex-situcharacterization of graphene. (a) Raman spectrum of graphene on Ag(111). (b) C1s XPS spectrum from region i without graphene and region ii–v with graphene. (c) O1s XPS spectrum from regions i and ii–v. Figure 3: Large-scale ex-situ characterization of graphene. ( a ) Raman spectrum of graphene on Ag(111). ( b ) C1s XPS spectrum from region i without graphene and region ii–v with graphene. ( c ) O1s XPS spectrum from regions i and ii–v. Full size image Ex-situ XPS was used to further characterize the graphene–Ag system. Although the XPS sampling area was not small enough to distinguish Fig. 1e–h , it was possible to isolate regions devoid of graphene ( Fig. 1d ) from areas containing graphene. Figure 3b shows the C1s spectra in regions i ( Fig. 1d ) and ii – v ( Fig. 1e–h ). It is clear that the 284.5 eV peak intensity is significantly increased from region i to region ii – v , indicating that the regions ii – v have a higher atomic C concentration. This result reaffirms the observation that a gradient in both carbon dose and graphene coverage exists across the sample. The O1s spectra also demonstrate noticeable dissimilarities, most obviously the large tail in the curve taken in regions ii – v . The asymmetry in Fig. 3c is explained by an increased ratio between the two peaks at 531.8 and 530.5 eV, which are commonly attributed to carboxyls and the electrophyllic oxygen state on Ag, respectively [39] . The strong increase in the peak at 531.8 eV in regions ii – v is attributed to the large portion of graphene edge states that interact with the oxidized/tarnished Ag surface after the sample is exposed to atmosphere. Finally, the decrease in the 530.5 eV peak from region i to regions ii – v suggests a decrease in Ag–O species that indicates that the graphene is protecting Ag from oxidation. Electronic characterization The electronic structure of the dendritic graphene was collected simultaneously with the topography via STS at energies of −200 and −60 meV, and is overlaid on a 3D rendering of the topography in Fig. 4a,b , respectively. Electronic scattering at the Ag surface state is visible as standing waves on the terraces in both images, clearly differentiating the Ag from graphene. At both energies, the graphene exhibits a distinct electronic structure near its edges: an enhanced electronic density of states (DOS) at −200 meV and a depressed DOS at −60 meV. The 3D topography illustrates that the differences in the dI / dV mapping are predominantly electronic in nature—dissimilar from the topographically raised edges observed in GNRs [40] , [41] . The edge state at −200 meV has a decay length of ~1.5–2 nm into the bulk graphene and generally exhibits a 30–50% DOS enhancement. Furthermore, the edge state observed in Fig. 3 is not only confined to the perimeter of the graphene flakes, but can be observed at grain boundaries in the graphene as well (highlighted in Fig. 4a ). Supplementary Fig. S3 shows the dispersion of the edge state from −1 to 1 V. The origin of the edge states observed here remains under investigation, but is currently thought to be unique to the Ag–graphene system, as they are not seen in the Cu–graphene system (under similar growth conditions). 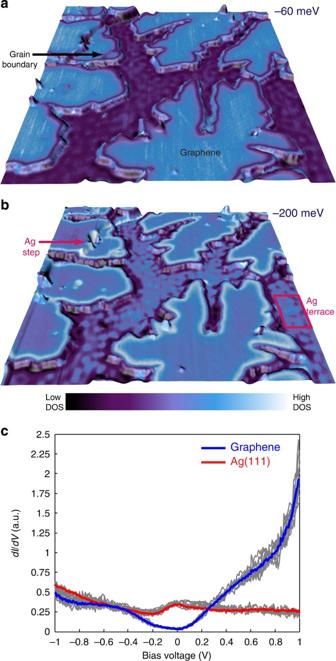Figure 4: Electronic characterization of graphene. (a) STS image collected at −200 meV superimposed on a 3D rendering of the underlying topography. (b) STS image collected at −60 meV of the same region pictured inasuperimposed on a 3D rendering of the underlying topography. Both images, 150 nm × 150 nm. (c)dI/dVpoint spectra for graphene and pristine Ag. Figure 4: Electronic characterization of graphene. ( a ) STS image collected at −200 meV superimposed on a 3D rendering of the underlying topography. ( b ) STS image collected at −60 meV of the same region pictured in a superimposed on a 3D rendering of the underlying topography. Both images, 150 nm × 150 nm. ( c ) dI / dV point spectra for graphene and pristine Ag. Full size image The dI / dV point spectra of the graphene and bare Ag(111) are shown in Fig. 4c . Notably, the surface state in the Ag spectrum appears near the Fermi level ( E f ); however, the Dirac point (DP) is not clearly visible in the graphene spectrum. Theoretical work has predicted electron transfer from Ag to graphene under equilibrium separation, which would set the DP at between −200 and −300 mV, similar to what is observed on Cu. Although the DP is not readily apparent, light doping is consistent with the slightly blue-shifted G-band in the Raman spectrum at ~1,589 cm −1 . In addition, the fact that the two materials differ significantly across the entire energy range provides strong evidence that the graphene is weakly coupled to the underlying substrate. In comparison, the electronic spectrum of graphene on Cu(111) is nearly identical to the clean Cu(111) spectrum [42] , with only a slight suppression of the Cu surface state. The electronic contrast between the two metal systems suggests a weaker binding of graphene on Ag than Cu, which is already considered to be in the weak binding regime [43] . Furthermore, the observation of several Moiré patterns indicates that the graphene is not in registry with the Ag lattice. Carrier scattering from graphene defects and edges has been predominantly studied on insulating substrates with the understanding that they are less perturbative to the electronic character of the graphene [18] , [19] . Previous work has established that intervalley backscattering is allowed only at armchair edges in graphene because of the limitations placed on the crystal momentum at the edges of the graphene [37] . This backscattering has been imaged via STM as a standing wave pattern at the edge of the graphene with a wavelength of λ f =2 π / k f =3a/2 on non-metallic substrates [18] , [19] and λ f /2 on a CVD copper foil [44] , where k f is the Fermi wavevector and λ f is the associated wavelength. The observed difference has been attributed to electronic confinement of the scattered waves to C–C bonds in the graphene on the insulators, whereas the confinement is absent on Cu because of the coupling between the graphene and Cu surface [18] , [44] . 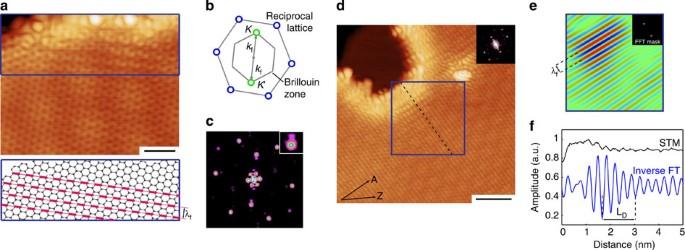Figure 5: Electronic scattering at graphene edges. (a) STM image of electronic scattering from a graphene edge (scale bar, 1 nm,V=25 mV,I=15 nA). Hexagonal lattice below gives suggested edge termination based on atomically resolved image; light pink lines indicate periodicity of the electronic interference with the thicker pink lines highlighting the C–C bonds where the charge is localized. (b)k-Space map of the 2D Fourier transform (FT) (c) of the image ina, showing the reciprocal lattice andK/K′ points. (d) Electronic backscattering from an armchair edge in the growth front with the lattice directions given in the lower left hand corner: A, armchair and Z, zig-zag (scale bar, 2 nm,V=25 mV,I=15 nA). Inset: 2D FT showing the RL andK/K′ points. (e) Inverse FT image of the boxed region fromdto highlight the spatial dependence of thekf(λf) scattering with the FT mask shown in the inset. (f) Height profile along the dashed line indicated indand corresponding profile of the inverse FT ine. Figure 5a illustrates a scattering pattern from a graphene edge on Ag, with the proposed edge termination given below. Clearly shown in both the STM and Fourier transform ( Fig. 5b,c ), the observed scattering has a wavelength (wavevector) of λ f ( k f ). Data collected from ~20 atomically resolved images yields λ f =3.62±0.13 Å, which is in good agreement with the theoretical prediction of λ f =3a/2=3.69 Å. This λ f quantum interference ( Fig. 5d ) also characteristically decays into the bulk graphene, consistent with previous observations [19] . A line profile ( Fig. 5f ) of the inverse Fourier transform shown in Fig. 5e displays a decaying profile away from the armchair edge with a decay length of L D =0.86±0.17 nm. Finally, a splitting of the k f scattering vector is shown in the inset to Fig. 5c , similar to the work on SiC, indicating the presence of long-range oscillations in the scattering envelope [18] . The presence of standing waves at graphene edges with periodicity λ f indicates that the DOS can be localized along the C–C bonds as on insulating substrates. Figure 5: Electronic scattering at graphene edges. ( a ) STM image of electronic scattering from a graphene edge (scale bar, 1 nm, V =25 mV, I =15 nA). Hexagonal lattice below gives suggested edge termination based on atomically resolved image; light pink lines indicate periodicity of the electronic interference with the thicker pink lines highlighting the C–C bonds where the charge is localized. ( b ) k -Space map of the 2D Fourier transform (FT) ( c ) of the image in a , showing the reciprocal lattice and K / K ′ points. ( d ) Electronic backscattering from an armchair edge in the growth front with the lattice directions given in the lower left hand corner: A, armchair and Z, zig-zag (scale bar, 2 nm, V =25 mV, I =15 nA). Inset: 2D FT showing the RL and K / K ′ points. ( e ) Inverse FT image of the boxed region from d to highlight the spatial dependence of the k f ( λ f ) scattering with the FT mask shown in the inset. ( f ) Height profile along the dashed line indicated in d and corresponding profile of the inverse FT in e . Full size image In conclusion, we report the successful growth of monolayer graphene on single-crystal Ag(111) under UHV conditions, using evaporated atomic carbon. The growth was conducted at relatively low substrate temperatures, making it a promising method for other low-melting-point substrates. The graphene growth was shown to emanate from small nanoparticles both at atomic steps and on terraces, generally leading to dendritic growth with large proportions of edges. The observation of quantum interference at the graphene edges highlights the weak interaction between the graphene and growth substrate. The ability to synthesize graphene on Ag in UHV opens the door to study interfaces with other 2D materials such as silicene. Graphene growth The Ag(111) crystal was cleaned with multiple cycles of Ar ion sputtering (1 kV, 10 −5 mbar) at room temperature, followed by annealing in UHV at 550 °C. Graphene growth was achieved through the deposition of elemental carbon onto a heated Ag(111) crystal at ~700 °C. The carbon was evaporated from a 99.999% pure graphite rod using a UHV e-beam evaporator; the sharpened carbon rod required an ~2 kV accelerating voltage and 30 mA emission current to sustain a consistent flux. On the basis of coverages estimated from STM images (all taken with a tungsten tip at 55 K), the deposition rate was well below 0.1 ML min −1 , in agreement with the negligible pressure changes observed during deposition (~10 −10 mbar). Carbon was deposited for 20 min, followed by immediate substrate cooling to room temperature. Scanning tunnelling microscopy STM microscopy was performed using an Omicron VT System with a base pressure of <10 −12 mbar. The experiments were conducted with electrochemically etched tungsten tips at ~55 K. STS was simultaneously collected by applying a small periodic modulation to the applied voltage and collecting the current with a SR830 Lock-In Amplifier. XPS was conducted in a Thermo Scientific ESCALAB 250 Xi at a base pressure of 10 −9 mbar. Raman spectroscopy was taken with a Renishaw InVia Raman Microscope System with a 514-nm laser line. How to cite this article: Kiraly, B. et al. Solid-source growth and atomic-scale characterization of graphene on Ag(111). Nat. Commun. 4:2804 doi: 10.1038/ncomms3804 (2013).